Taller plants have lower rates of molecular evolution Rates of molecular evolution have a central role in our understanding of many aspects of species’ biology. However, the causes of variation in rates of molecular evolution remain poorly understood, particularly in plants. Here we show that height accounts for about one-fifth of the among-lineage rate variation in the chloroplast and nuclear genomes of plants. This relationship holds across 138 families of flowering plants, and when accounting for variation in species richness, temperature, ultraviolet radiation, latitude and growth form. Our observations can be explained by a link between height and rates of genome copying in plants, and we propose a mechanistic hypothesis to account for this—the ‘rate of mitosis’ hypothesis. This hypothesis has the potential to explain many disparate observations about rates of molecular evolution across the tree of life. Our results have implications for understanding the evolutionary history and future of plant lineages in a changing world. Many factors have been proposed to drive rates of molecular evolution in plants, including environmental energy, water availability, temperature, ultraviolet (UV) radiation, speciation rate, generation time and metabolic rate [1] , [2] , [3] , [4] , [5] , [6] , but disentangling these factors has been difficult. The results of many studies are equivocal or contradictory and there is confusion over the way in which some proposed mechanisms, especially the generation time effect, may operate [1] . Indeed, the vast majority of variation in rates of molecular evolution among plants remains both unexplored and unexplained. Body size is fundamentally important to multiple aspects of the ecology, physiology and evolution of both animals and plants [7] , [8] , [9] , [10] . Because of this, analysing and understanding the relationship between body size and rates of molecular evolution has led to many important discoveries in animals [10] . However, the link between body size and rates of molecular evolution has not been examined in plants, despite its potential to elucidate many important but poorly understood aspects of plant molecular evolution. Here, we use sister pairs and phylogenetically corrected linear regressions [11] to test for associations between rates of molecular evolution, height and other aspects of plant biology. Our results demonstrate that taller families of plants tend to have slower rates of molecular evolution in both the chloroplast and nuclear genomes. Furthermore, the association between height and rates of molecular evolution holds when accounting for variation in species richness, UV, temperature and latitude, and is also significant when considering exclusively herbaceous plant families, or those that contain only shrubs and trees. We discuss four possible mechanisms that might cause an association between rates of molecular evolution and height in plants: generation time, metabolic rate, population size and rates of mitotic cell division in the apical meristem. We conclude that metabolic rate and population size are unlikely to contribute to the association between rates and height, but that generation time and rates of mitosis may do so. This is because taller families of plants may comprise species with both longer generation times (and thus slower long-term rates of meiosis) and slower long-term rates of mitosis in their apical meristems. Data sets We assembled a data set of 138 families of flowering plants, grouped into 69 sister pairs. For each family, we estimated the amount of genetic change for the chloroplast and nuclear genomes from a large DNA sequence data set [12] . We estimated molecular branch lengths in substitutions per site, and absolute rates of molecular evolution in substitutions per site per million years. We did this using maximum-likelihood methods corrected to account for a known bias in branch length estimation (the node density effect; see Methods). We also estimated the average maximum height of the species in each family, using a database of maximum plant height records for over 20,000 species [13] collected to describe global patterns in plant height. Sister pairs analyses In our study, a sister pair comprises two families of plants that share a common ancestor to the exclusion of all other families in our data set. Both families are therefore the same age, and have had the same amount of time to accrue genetic differences. Consequently, any difference in the amount of genetic change that the two families have accumulated represents a difference in the underlying rate of molecular evolution, and differences in rates of molecular evolution can be calculated without knowing, or estimating, divergence dates of the sister pairs [11] . Across all sister pairs, two distinct statistical tests indicate a significant association between the average maximum height a family and the rate of molecular evolution of that family. Two-tailed sign tests on sister pairs demonstrate that the taller plant family within each pair has the shorter branch length more often than expected by chance for both the chloroplast ( P =0.024) and nuclear genome ( P =0.005). Linear regressions of differences in height versus differences in branch lengths calculated from sister pairs confirm the significance of these associations and quantify their magnitude: height accounts for 16% of the variation in synonymous rates of molecular evolution in the chloroplast genome ( B =–0.17, P =0.001; Fig. 1a ) and 25% of the variation in rates of molecular evolution in nuclear rRNAs ( B =–0.28, P =4 × 10 −5 ; Fig. 1b ). 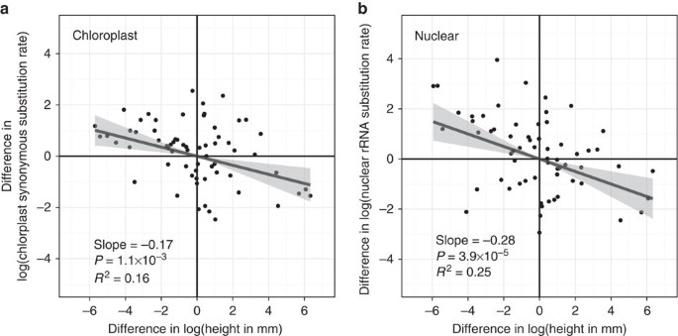Figure 1: The relationship between plant height and rates of molecular evolution in angiosperms. Differences in the logarithms of plant height and rates of molecular evolution were measured for sister pairs of angiosperm families. Regressions through zero show a significant negative association between plant height and synonymous substitution rates measured from protein-coding genes in the chloroplast genome (a), and between plant height and substitution rates in rRNA genes in the nuclear genome (b). In each panel, the best-fit line (dark grey) was estimated using linear regression through the origin, with the 95% confidence intervals around this line shown in light grey (see main text). Figure 1: The relationship between plant height and rates of molecular evolution in angiosperms. Differences in the logarithms of plant height and rates of molecular evolution were measured for sister pairs of angiosperm families. Regressions through zero show a significant negative association between plant height and synonymous substitution rates measured from protein-coding genes in the chloroplast genome ( a ), and between plant height and substitution rates in rRNA genes in the nuclear genome ( b ). In each panel, the best-fit line (dark grey) was estimated using linear regression through the origin, with the 95% confidence intervals around this line shown in light grey (see main text). Full size image Sister pairs analyses accounting for other variables To better understand the link between height and rates that we have observed, we assessed whether the relationship was affected by other known correlates of rates of molecular evolution in plants. In total, we were able to calculate family-level estimates of species richness, temperature, levels of UV radiation and latitude, each of which has been linked to rates of molecular evolution in previous studies [2] , [3] , [4] . We estimated differences in each of these variables for each of the sister pairs in our analysis and re-evaluated the relationship between height and molecular rates, including these additional variables as covariates (see Methods). We used the sister-pairs approach for these analyses because it makes the fewest assumptions of the available comparative methods about the ways in which rates and traits change over time [11] . We estimated all pairwise models including height and each of the other variables as predictors of molecular rates in both the chloroplast and nuclear genomes ( Tables 1 and 2 , respectively). We also estimated the full model including all variables as predictors of molecular rates in the chloroplast and nuclear genomes ( Fig. 2 , Tables 3 and 4 ), and models including each of the additional variables as a predictor of height. Table 1 Pairwise regressions of chloroplast synonymous substitution rates. 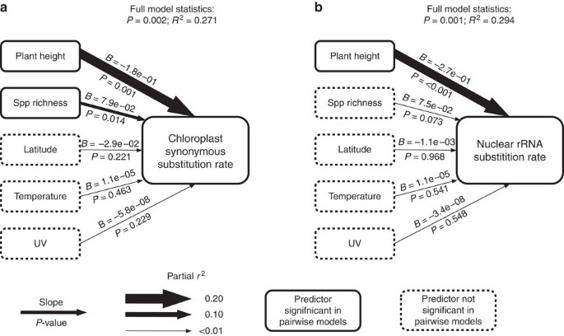Figure 2: Biological predictors of rates of molecular evolution in plants. Five potential predictors of substitution rates were measured for each plant family, log-transformed and included in two different linear models: (a) synonymous substitution rates in chloroplast protein-coding genes; and (b) substitution rates in nuclear rRNA genes. TheP-value andR2of the full model are shown above each diagram. The width of each arrow represents the partialr2of each predictor, which estimates the effect of that predictor after controlling for all other predictors. The slope and significance of each predictor are shown above and below each arrow, respectively. Predictors that were significant in pairwise linear models with plant height are shown in solid boxes, and those that were not significant are shown in dashed boxes. Plant height was significant in all pairwise linear models (Tables 1and2). Full size table Table 2 Pairwise regressions of nuclear rRNA substitution rates. Full size table Figure 2: Biological predictors of rates of molecular evolution in plants. Five potential predictors of substitution rates were measured for each plant family, log-transformed and included in two different linear models: ( a ) synonymous substitution rates in chloroplast protein-coding genes; and ( b ) substitution rates in nuclear rRNA genes. The P -value and R 2 of the full model are shown above each diagram. The width of each arrow represents the partial r 2 of each predictor, which estimates the effect of that predictor after controlling for all other predictors. The slope and significance of each predictor are shown above and below each arrow, respectively. Predictors that were significant in pairwise linear models with plant height are shown in solid boxes, and those that were not significant are shown in dashed boxes. Plant height was significant in all pairwise linear models ( Tables 1 and 2 ). Full size image Table 3 Multiple regression of chloroplast synonymous substitution rates. Full size table Table 4 Multiple regression of nuclear rRNA substitution rates Full size table In all cases, height remained a significant predictor of molecular rates and consistently explained around one-fifth of the variation in rates of molecular evolution in both the chloroplast and nuclear genomes ( Fig. 2 , Tables 1 , 2 , 3 , 4 ). We also found a marginally significant ( P =0.068) negative association between height and latitude, and a significant ( P =0.025) positive association between height and temperature (see also ref. 13 ). Weighted sister-pairs analyses We performed weighted linear regressions to attempt to account for the differences in variance associated with our family-level height estimates (see Methods). The results of these analyses are qualitatively identical to the unweighted regressions. In linear models comparing height to rates of molecular evolution, weighted regressions show a significant negative association between height and rates of molecular evolution, and suggest that height accounts for 11–27% of the variation in rates of molecular evolution (chloroplast genome: B =–0.17, P =0.005, R 2 =0.11; nuclear genome: B =–0.29, P =9 × 10 −6 , R 2 =0.27). Similarly, weighted regressions of the full model including five predictors of rates of molecular evolution (height, species richness, latitude, temperature and UV) showed a significant negative correlation between height and the rate of molecular evolution in the chloroplast ( B =–0.18, P =0.004) and nuclear genomes ( B =–0.29, P =3 × 10 −5 ). As with the unweighted regressions, all other predictors were nonsignificant except for species richness, which was significantly positively correlated to the rate of molecular evolution in the chloroplast genome ( P =0.047). Phylogenetic generalized least-squares analyses of height and rates of molecular evolution It is also possible to analyse the relationship between height and rates of molecular evolution by estimating the absolute rate of molecular evolution (in substitutions per site per million years) for each of the 138 families of plants in our data set (see Methods). This approach makes additional assumptions about the way that rates of molecular evolution change over time, and about the divergence dates of each of our sister pairs [11] . But it also provides more statistical power than a sister-pairs analysis, and allows us to straightforwardly account for uncertainty in the phylogenetic tree and molecular rate estimates using non-parametric bootstrapping (see Methods). We used phylogenetic generalized least-squares (PGLS) regressions to compare log-transformed height to log-transformed absolute rates of molecular evolution, calculated from the combined nuclear and chloroplast data set. These analyses reveal highly significant negative associations between height and overall rates of molecular evolution ( B =–0.05, P =3 × 10 −7 , R 2 =0.41). These relationships hold when accounting for uncertainty in the phylogeny and molecular rate estimates using 1,000 non-paramteric bootstrap replicates (see Methods)—the 95% bootstrap confidence interval of the R 2 value is 0.33–0.48, the 95% confidence interval of the slope is −0.04 to −0.06, and all 1,000 bootstrap replicates were statistically significant. The results are qualitatively identical when using weighted PGLS regressions. Analyses of herbaceous and woody plant families Previous studies have suggested that herbaceous and woody species show significantly different rates of molecular evolution [6] . Because of this, we conducted separate PGLS analyses for those families in our data set that are exclusively herbaceous ( n =25) and those that comprise only trees and/or shrubs ( n =60). In both cases, we observed significant negative associations between height and overall rates of molecular evolution calculated from the combined data set (herbs: B =–0.10, P =0.003, R 2 =0.25; trees/shrubs: B =−0.05, P =0.019, R 2 =0.07). Our results demonstrate that taller families of plants evolve more slowly than shorter families, and that this association is independent of many other known correlates of rates of molecular evolution including temperature, latitude, UV radiation and species richness. The association between height and rates of molecular evolution holds for both the nuclear and chloroplast genomes, and across families that contain exclusively herbaceous species, as well as those that contain exclusively shrubs and trees. Our results are also robust to uncertainty in the underlying phylogenetic tree topology and molecular rate estimates. The strength of the association between height and rates of molecular evolution is particularly striking because our family-level estimates of both height and rates of molecular evolution are necessarily crude due to incomplete sampling. Taking averages of traits for families of plants overlooks the fine-scale variation in traits that may occur between closely related species, and ignores the sometimes substantial variation among traits and rates within families. These factors are expected to introduce significant random error into our analysis, which suggests that the association between height and rates of molecular evolution may be even stronger than we have been able to detect in this study. What might explain an association between height and rate of molecular evolution in plants? We consider four possible mechanisms below: generation time, metabolic rate, population size and rates of mitotic cell division in the apical meristem. If taller families of plants tend to comprise species with longer generation times, our results could be explained by the effects of generation time on mutation or fixation rates in plant genomes. The generation time hypothesis states that species with shorter generation times copy their genomes more often, and consequently accrue more replication errors per unit time, resulting in higher mutation rates [14] . The generation time hypothesis assumes that generation time is correlated with the overall rate of genome replication. This is unlikely to be strictly true for plants because they grow from apical meristems, which undergo continual mitosis and from which reproductive tissues are derived late in development. Because of this, the number of mitotic cell divisions in plants can vary substantially between generations and among closely related species [15] . In contrast, many animals have deterministic development in which there is a fixed number of mitotic cell divisions in each generation. As a result, generation time can provide a useful proxy of the overall rate of genome replication in animals, but is unlikely to do so in plants. This may explain why the evidence for the generation time hypothesis is very strong for animals [16] , [17] , [18] , but mixed for plants [1] , [19] , [20] , [21] . Despite this, generation time will remain tightly associated with long-term rates of meiosis in plants, because an extant plant genome would have experienced one meiosis in each generation through which it has passed. Therefore, if a significant proportion of heritable mutations are associated with meiosis in plants, and if taller families of plants tend to have longer generation times, then a generation time effect on mutation rates might explain our results. A generation time effect on substitution rates could also explain our results, because all else being equal, generation times determines the absolute timescale of genetic drift. The metabolic rate hypothesis proposes that organisms with higher mass-specific metabolic rates produce a higher concentration of damaging metabolic by-products (oxygen radicals), and thus accumulate more DNA damage and more mutations per unit time [22] . The metabolic rate hypothesis could explain our results if taller plants have lower mass-specific metabolic rates in their apical meristems. Although this is possible [9] , allometry theory predicts, and empirical data show, that cellular metabolic rates of certain tissues are essentially independent of plant height [23] , undermining a potential role for metabolic rate in driving rates of molecular evolution in plants. Furthermore, although correlative evidence for the metabolic rate hypothesis in animals is mixed [24] , [25] , [26] , experiments in animals have shown that oxygen radicals generated in organelles do not damage the nuclear DNA of the same cell [27] , and that germ-line mutations do not accumulate under increased oxidative stress [28] . If the same is true for plants, the metabolic rate hypothesis cannot explain the link we have observed between height and rates of molecular evolution in the nuclear genome. If taller families of plants tend to comprise species with larger effective population sizes ( N e ), and if a significant proportion of the genomic changes we have measured are deleterious, then a population size effect could explain our results. In this case, selection would be more effective in taller plants, and so slightly deleterious mutations would be fixed less frequently in these lineages [29] . If taller plants have larger N e , we would expect a negative correlation between height and the ratio of non-synonymous to synonymous substitutions (d N/ d S [29] ). To test this prediction, we compared differences in d N/ d S to differences in height across all of our sister pairs. We found that height was significantly positively correlated to d N/ d S ( B =0.16±0.07, P =0.02, R 2 =0.08). This suggests that taller plants have smaller N e and does not support a population size effect as an explanation for our results. To account for the possibility that rates of mitosis could drive rates of molecular evolution in plants, we propose a novel explanation for our results here—the ‘rate of mitosis’ (ROM) hypothesis. The ROM hypothesis states that a substantial fraction of mutations that accumulate in the germ-line DNA of plants occur during mitotic cell divisions in the apical meristem. Such mutations are potentially heritable because plants do not sequester their germ lines until very late in development [30] , [31] . Thus, species with higher rates of mitotic cell division in the apical meristem will copy their DNA more frequently, accrue more DNA replication errors per unit time, and have higher rates of mutation and substitution. Crucially, the long-term rate of mitosis in the apical meristem is likely to be lower in taller plants, because growth slows as plants increase in size and because there are physical limits to the delivery of water and nutrients to apical meristems as they increase in distance from the root system [1] , [9] , [20] , [32] , [33] , [34] . Thus, the ROM hypothesis predicts that taller plants will have lower mutation rates, potentially explaining the observations we have made in this study. Interestingly, the ROM hypothesis could help to explain many other observations about rates of molecular evolution in plants and animals. For example, it can explain why perennials evolve more slowly than annuals, why woody plants evolve more slowly than herbs and why tree ferns evolve more slowly than other ferns [1] , [6] , [35] . In all three of these cases, the faster-evolving plants (annuals, herbs and non-arborescent ferns) are likely to have higher rates of mitosis than their more slowly evolving relatives (perennials, woody species and tree ferns), although we also note that the faster-evolving plants are also likely to have shorter generation times in all of these cases. The ROM hypothesis might also explain why generation times correlate with rates of molecular evolution in animals, but not in plants [20] , [21] , [36] , because generation times are a reliable predictor of rates of mitosis in animals, but not in plants. Finally, the ROM hypothesis might explain previously observed correlations between rates of molecular evolution and environmental energy [3] , latitude [2] and water availability [5] in plants. In all three of these cases, the faster-evolving taxa are associated with conditions more favourable for rapid plant growth (higher environmental energy, latitudes close to the tropics and higher water availability). Higher growth rates are likely to be associated with higher rates of mitosis in the apical meristem, and therefore with higher rates of mutation and substitution. It is not possible from our data to distinguish the relative contributions of meiosis and mitosis to rates of molecular evolution in plants. However, this may be possible in systems where long-term rates of meiosis are constant across species, such as between closely related annual plants. In this case, the ROM hypothesis predicts that taller annual plants have higher rates of molecular evolution (the opposite to the pattern shown here) because their apical meristems will undergo more mitotic cell divisions per year. Thus, comparing the rates of molecular evolution to height in closely related annual plants may provide a useful test of the ROM hypothesis, and may allow future studies to more directly assess the relative contributions of meiosis and mitosis to rates of molecular evolution in plants. Our results further underline the central role of height in the ecology and evolution of plants. We have shown that taller plants have lower rates of molecular evolution than shorter plants, and that this is likely to be driven by lower underlying mutation rates caused by lower rates of genome copying in taller plants. This has implications for reconstructing the evolutionary history of plants using techniques such as molecular dating, because it informs our expectations of rate variation among plant lineages. It also has implications for predicting the evolutionary future of plants, because the ability of species to adapt to a changing world depends critically on their underlying mutation rates [37] . Phylogeny estimation and selection of sister pairs We estimated a phylogenetic tree of flowering plants using the DNA data set of Burleigh et al. [12] , comprising 567 species and 10,552 base pairs. We refined their alignments [12] , then partitioned the data set into MatK (which is often a pseudogene), 1st+2nd codon positions, 3rd codon positions, RNA stems and RNA loops. We estimated a maximum-likelihood topology using RaxML [38] , applying an independent GTR+I+G model to each data partition. We then assigned each species in the tree to a family of plants [29] , [39] , and retained only those families that were recovered as monophyletic in our tree. Finally, we chose all sister pairs of monophyletic families in our tree for our final analysis, resulting in a data set of 138 monophyletic angiosperm families grouped into 69 sister pairs ( Fig. 1 ). Input and output files for RAxML are available from DataDryad. Branch length estimation The sister-pairs method requires that branch lengths be estimated for each family of each sister pair. The more species from a family that can be included in each branch length estimate, the more representative that branch length estimate will be as an estimate of the branch length of the family in question. However, branch length estimation suffers from a known bias, whereby longer branch lengths tend to be inferred in clades with higher node density [40] . In our case, this could create an artefactual association between species richness and molecular branch lengths. To avoid this, we first equalized the number of representative species of the two members of each sister pair, by randomly deleting species from the family with more representative species. This ensures that the branch lengths for each sister pair are calculated from families with equal node density, thus removing the node density artefact from our data [11] . The removal of species in this way increases the variance of our branch lengths as estimators of the branch length of a given family of plants, but serves to remove any biases in these estimators. Thus, this method reduces the power of our approach to detect associations between rates of molecular evolution and traits such as height. This resulted in a tree of 196 taxa, with the majority of sister pairs comprising families represented by a single species in the tree (49/69 sister pairs), and the remaining sister pairs comprising families represented by two to four species per family. Using this tree of 196 taxa, we estimated branch lengths using maximum-likelihood in HyPhy v2.0 (ref. 41 ). For families with more than one representative in our data set, we calculated the phylogenetic average of the family branch lengths by successively averaging branch lengths down the phylogeny for each family [4] . The result of this was an estimate of the nuclear ribosomal RNA and chloroplast synonymous branch lengths for each of the 138 families in our data set. These data are available from DataDryad. Estimation of absolute rates of molecular evolution We estimated absolute rates of molecular evolution in substitutions per site per million years across the entire 10,552-bp alignment using R8s [42] . To do this, we first selected at random one representative species from each of the 140 families in our data set for which we had height estimates, in order to avoid the node density effect in our rate estimations (138 families from sister pairs, plus two additional families which we excluded from the sister-pair analyses because they did not fall into sister pairs). We then used RAxML [38] to calculate the ML tree with branch lengths from the 10,552-bp, 140 taxon data set, as well as 1,000 bootstrap trees with branch lengths using non-parametric bootstrapping. We then used a Python script to calculate absolute rates of molecular evolution on each of the trees using a diverse set of 30 fossil calibrations [43] . This script and the input and output from R8s are available from DataDryad. Estimation of average maximum height for each family To calculate the average maximum height for each of the 138 families in our data set, we used a published database of over 32,737 maximum plant height records from 20,679 species [13] . This data set has been rigorously curated to ensure that taxonomic names are accurate, that synonyms are accounted for, that extreme values in the data set are legitimate and that all measurements represent maximum recorded height from a published source [13] . To calculate the average maximum height for each family, we first calculated the arithmetic mean of the log-transformed maximum heights of each genus in the family. We then calculated the arithmetic mean of the genus-level averages to provide an estimate of the average maximum height of each family. We are unable to release the raw height data set from Moles et al. [13] , because this would violate several data-sharing agreements, however, the family average height data on which the analyses in this study are based are available on DataDryad. Using phylogenetic averaging in this way ensures that our estimates of plant height are, to the best of our ability, comparable to our estimates of molecular branch lengths. This is because branch length estimates represent the integral of the rate of molecular evolution over the entire history of a lineage, rather than an estimate of the rate of molecular evolution in the present day. On the other hand, traits such as plant height are measured exclusively from extant taxa. A phylogenetic average of a trait represents a measure of central tendency that is more comparable to the estimates of molecular rates that we use, and this approach has been shown to improve the power of comparative studies of molecular rate variation [44] . Our estimates of plant height will in many cases be associated with high variance, particularly where our sampling of the extant taxa in a family is sparse, and/or the variance in height within a given family is large. This will introduce noise, but not bias, into our analysis, because the sampling of plant heights in the data set is not biased with respect to the rates of molecular evolution of the plants in question. To attempt to account for this sampling variance, we performed weighted regressions in which we used as weights the proportion of extant genera in each sister pair (for sister pairs analyses) or family (for PGLS analyses) for which we had at least one height record. Thus, the more of the extant genera we have sampled for a given sister pair or family, the higher the weight of that data point in the regression. We use the proportion of genera because genus-level sampling will have the largest effect on our phylogenteically averaged height estimates. Using these weights may help to account for the different variances associated with our height estimates, although we acknowledge that the approach is far from perfect. Estimation of other traits for each family Species numbers in each family were estimated from the Families of Flowering Plants database ( http://delta-intkey.com ) following Barraclough et al. [4] , as were the existence of species in each family that were herbs, shrubs or trees. All other variables (latitude, UV irradiation and temperature) were estimated by calculating the mean value of each trait per unit of area using digital distribution maps for each family of plants [3] . Trait data is available from DataDryad. Diagnostic tests on the data Parametric analyses (such as linear models) of sister pairs make certain assumptions about the data. To ensure that these assumptions were met, we performed three diagnostic tests on the differences in rates and traits that we calculated, following the advice given in Lanfear et al. [11] . These comprise: (i) a test to check that our log transformation of all rates and traits removed any association between the variance of data points and their absolute values [45] ; (ii) a test to ensure that variance in rate and trait differences increases linearly with evolutionary time [46] ; and (iii) a test to ensure that the variance in rate differences was not affected by low numbers of substitutions [44] . The first test indicated that log transformations of rate and trait data were appropriate for most traits and rates, except temperature and UV which were squared, and latitude which was left untransformed. The second test indicated that standardizing all differences by the square root of the sum of the branch lengths (as suggested in ref. 46 ) in each sister pair was appropriate. The third test indicated that four of the sister-pair differences in chloroplast synonymous branch lengths were unreliable (leaving a total of 65 sister pairs with reliable data), and that six of the sister-pair differences in nuclear rRNA branch lengths were unreliable (leaving 63 sister pairs with reliable data). Accordingly, we performed all statistical tests with and without these unreliable sister pairs, and the results are qualitatively identical in all cases. The results reported here are those with the unreliable data points removed, which is the approach suggested in previous studies [11] , [44] . Statistical analysis All statistical analyses were performed in R [47] . For the sister-pairs data, we performed linear regressions through zero [46] of the transformed trait data, after excluding sister pairs for which rate estimates were unreliable. The slope, s.e. of the slope and P -values for each variable in linear regressions were calculated using the lm() function in R. Partial correlation coefficients (partial r ) and partial coefficients of determination (partial r 2 ) were calculated in R using matrix inversion of pearson correlations between pairs of variables. For the absolute rate analyses, we performed PGLS regression using the CAPER and nlme packages. Analyses on the ML tree using CAPER indicated that the best fit of the model to the data was obtained when optimizing the ‘delta’ parameter during the PGLS. Therefore, we performed all PGLS analyses by optimizing ‘delta’. R scripts are available from DataDryad. Data availability All data, including data on trees, traits, rates, fossil calibrations, R code and Python scripts used for this publication are available from DataDryad at http://dx.doi.org/dryad.43mg3 . How to cite this article: Lanfear, R. et al. Taller plants have lower rates of molecular evolution. Nat Commun. 4:1879 doi: 10.1038/ncomms2836 (2013).